Porous covalent electron-rich organonitridic frameworks as highly selective sorbents for methane and carbon dioxide Carbon dioxide capture from point sources like coal-fired power plants is considered to be a solution for stabilizing the CO 2 level in the atmosphere to avoid global warming. Methane is an important energy source that is often highly diluted by nitrogen in natural gas. For the separation of CO 2 and CH 4 from N 2 in flue gas and natural gas, respectively, sorbents with high and reversible gas uptake, high gas selectivity, good chemical and thermal stability, and low cost are desired. Here we report the synthesis and CO 2 , CH 4 , and N 2 adsorption properties of hierarchically porous electron-rich covalent organonitridic frameworks (PECONFs). These were prepared by simple condensation reactions between inexpensive, commercially available nitridic and electron-rich aromatic building units. The PECONF materials exhibit high and reversible CO 2 and CH 4 uptake and exceptional selectivities of these gases over N 2 . The materials do not oxidize in air up to temperature of 400 °C. Flue gas emitted from coal-fired power plants constitutes 15–16% CO 2 , 6–7% H 2 O, 3–4% O 2 , and about 70% N 2 (ref. 1 ). Carbon dioxide capture from coal-fired power plant emitters is currently considered as a possible technology to stabilize the CO 2 level in the atmosphere to avoid climate changes [2] . A variety of sorbent materials are currently under investigation for carbon dioxide capture. The key features of suitable sorbents for carbon dioxide capture are high selective uptake of CO 2 , facile regeneration of the sorbent at low-energy penalty, low cost of the sorbent material, chemical stability towards H 2 O, O 2 , SO x , and NO x , as well as good thermal stability. Porous materials have been discussed as promising sorbents for carbon dioxide capture. Several classes of porous materials are currently under investigation, predominantly metal–organic frameworks (MOFs) [3] , [4] , [5] , [6] , [7] , [8] , [9] , [10] , [11] , activated carbons [12] , [13] , [14] , molecular organic solids [15] , and amine-functionalized silicas [16] , [17] , [18] , [19] , [20] . More recently, also reports on CO 2 sorption in porous covalent organic frameworks and polymers have been published [21] , [22] , [23] , [24] . Generally, sorbents which physisorb CO 2 (for example, MOFs and carbons) tend toward lower selectivity and gas uptake at low CO 2 pressure (≤1 atm) but exhibit facile reversibility, while strongly chemisorbing materials such as amine-functionalized silicas tend towards higher selectivities and capacities but typically show less facile reversibility. Recently, amine-functionalized MOFs have been reported that exhibit increased CO 2 sorption at low pressure as well as significantly improved selectivity [4] , [5] . Still, MOFs tend toward chemical instability (oxidation, hydrolysis) due to the dative nature of the metal–ligand bonds. It is apparent that sorbents with enhanced chemical stabilities and heats of adsorption at the borderline between strong physisorption and weak chemisorption (ca. 25–50 kJ mol −1 ) are an attractive target to reach a good trade-off between selectivity and reversibility. Here we produce novel porous electron-rich covalent organonitridic frameworks (PECONFs) as potential sorbents for carbon capture. In PECONFs, inorganic nitridic building units are interconnected via electron-rich aromatic units to form porous covalent frameworks. Carbon dioxide sorption is expected to occur because of the Lewis-acid Lewis-base interactions between the electron-rich aromatic constituents and the electron-poorer carbon dioxide molecules. In addition, weak Lewis acid-base interactions between the lone pairs at the nitridic building units and CO 2 could contribute. Both types of interactions are likely stronger than simple dispersion forces (5–20 kJ mol −1 ) but weaker than strong chemisorptive interactions (>50 kJ mol −1 ), because no covalent bonds are formed between the sorbent and CO 2 . The covalent and inert nature of the bonds in PECONFs suggests high chemical stability. Synthesis We have produced archetypes of porous electron-rich covalent organonitridic frameworks (PECONFs) from inexpensive 3,3′-diaminobenzidine (DAB) and hexachlorocyclotriphosphazene ( Fig. 1 ) in simple polycondensation reactions using dimethylsulphoxide (DMSO) as the solvent. DAB acts as the electron-rich aromatic building block [25] , [26] , [27] due to its four amino groups while hexachlorocyclotriphosphazene has the role of the nitridic building unit. These building blocks are significantly less expensive than those used for covalent organic frameworks and polymers typically used so far [21] , [22] , [23] , [24] . The materials were obtained as monoliths, which could be solvent-exchanged and dried without cracking or disintegration ( Supplementary Fig. S1 ). The microstructures of the monoliths could be modulated by systematically decreasing the amount of the solvent (DMSO) in the reaction mixture (see Supporting Information ). 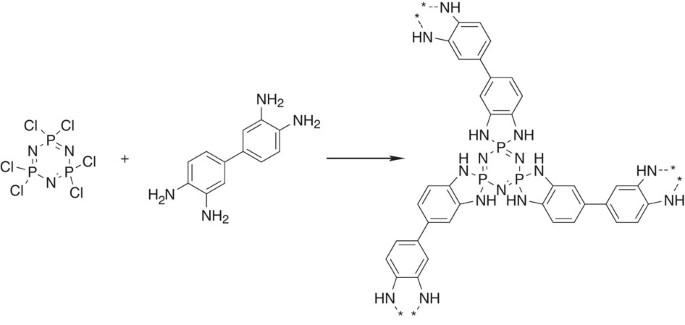Figure 1: Reaction scheme for the synthesis of PECONFs. Hexachlorocyclotriphosphazene and diaminobenzidine react in polycondensation reactions from DMSO solutions to form PECONF materials. Figure 1: Reaction scheme for the synthesis of PECONFs. Hexachlorocyclotriphosphazene and diaminobenzidine react in polycondensation reactions from DMSO solutions to form PECONF materials. Full size image Electron microscopy and X-ray diffraction The scanning electron microscopy (SEM) ( Fig. 2 ) and transmission electron microscopy (TEM) ( Supplementary Fig. S2 ) images of the PECONFs show that the materials are composed of intergrown, nearly spherical particles. The diameter of the spheres is a function of the reactant concentration. PECONF-1, which was synthesized at the highest concentrations, showed the largest spheres with diameters around 600 nm. PECONF-2 and PECONF-3, which were synthesized at decreased reactant concentrations, exhibited decreased sphere diameters of around 400 and 200 nm, respectively. The moderate intergrowth of the spheres produced macropores between the spheres. PECONF-4, which was prepared at the lowest reactant concentrations, has a polygranular structure with grain sizes in the order of a few tens of nanometers. As a consequence, PECONF-4 does not exhibit macroporosity. All materials were non-crystalline, according to powder X-ray diffraction ( Supplementary Fig. S3 ) and selective area electron diffraction ( Supplementary Fig. S4 ). 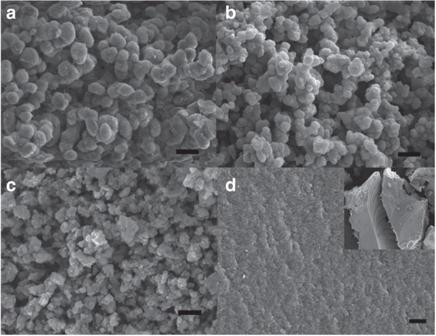Figure 2: Scanning electron microscopy images of PECONFs. (a) PECONF-1, (b) PECONF-2, (c) PECONF-3, and (d) PECONF-4. PECONF-1, 2, and 3 exhibit macroporous structures of weakly intergrown spherical particles with tunable diameters. PECONF-4 does not show any macroporosity. Scale bar equals one micrometer. Figure 2: Scanning electron microscopy images of PECONFs. ( a ) PECONF-1, ( b ) PECONF-2, ( c ) PECONF-3, and ( d ) PECONF-4. PECONF-1, 2, and 3 exhibit macroporous structures of weakly intergrown spherical particles with tunable diameters. PECONF-4 does not show any macroporosity. Scale bar equals one micrometer. Full size image MAS NMR spectroscopy To investigate the structure of the materials in more detail, we have studied the 31 P MAS NMR and 13 C CP MAS NMR spectra of the PECONFs. 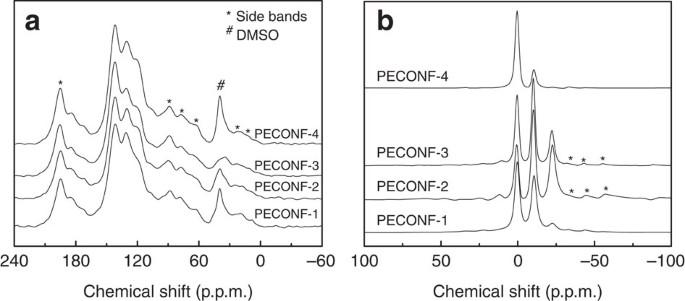Figure 3: Cross-polarization magic angle spinning nuclear magnetic resonance (CPMAS NMR) of PECONFs. (a)13C CPMAS NMR spectra and (b)31P CPMAS NMR spectra of PECONF-1, PECONF-2, PECONF-3, and PECONF-4 are in accordance with structures composed of interconnected cyclotriphosphazene and diaminobenzidine building blocks. Side bands are indicated by a star. Figure 3a shows the 13 C spectra of PECONFs. Strong signals around 141 and 131 p.p.m. with a shoulder at 121 p.p.m. and a small weak signal at 106 p.p.m. were observed in the 13 C CP MAS spectra. The chemical shifts are consistent with the presence of the DAB building block. This confirms that the electron-rich aromatic DAB unit was incorporated into the PECONF materials. An additional signal was observed around 39 p.p.m., which can be assigned to residual DMSO that was used as the solvent for the synthesis. Figure 3: Cross-polarization magic angle spinning nuclear magnetic resonance (CPMAS NMR) of PECONFs. ( a ) 13 C CPMAS NMR spectra and ( b ) 31 P CPMAS NMR spectra of PECONF-1, PECONF-2, PECONF-3, and PECONF-4 are in accordance with structures composed of interconnected cyclotriphosphazene and diaminobenzidine building blocks. Side bands are indicated by a star. Full size image The 31 P MAS NMR spectra ( Fig. 3b ) of the PECONFs showed signals in the range from 0 to −25 p.p.m. which are typical for P(V)N 4 tetrahedra [25] , [26] , [28] . In PECONF-1, two strong, and one weak signal were observed at 0.4, −10.4, and −22.5 p.p.m., respectively. In PECONF-2, 3, and 4 three signals at almost identical chemical shifts were seen. All the signals were astonishingly sharp given that all the materials were non-crystalline indicating a comparatively high degree of order. The observation of three signals suggests that three different phosphorus environments are present in the frameworks. This may be explained by the fact the P atoms can be surrounded by bridging as well as terminal DAB units in the framework. Fourier transform infrared spectroscopy The PECONF materials were further studied by Fourier transform infrared spectroscopy ( Supplementary Fig. S5 ). All the spectra show a broad band around 3,420 cm −1 and a sharp band around 1,617 cm −1 . These bands can be attributed to the N–H stretching and bending vibrations, respectively. Furthermore, several broad bands are observed in the region from 1,500 to 500 cm −1 . The bands at ~1,090 and ~950 cm −1 can be attributed to the ν as (P–NH–P) vibrations. The bands at 1,218 and 1,420 cm −1 are due to the ν as (P=N–P) vibrations. The band around 520 cm −1 can be assigned to the δ(P=N–P) vibrations. Similar bands are also observed in phosphorus nitride, nitride imides, and oxynitrides [29] , [30] , [31] , [32] , [33] . The sharpness of the bands in the fingerprint region suggests a relatively high degree of order in the materials which corroborates the results from 31 P MAS NMR spectroscopy. Thermal and chemical properties We further studied the thermal behaviour and the oxidative stability of the PECONFs. Supplementary Figure S6 shows the thermogravimetric analysis (TGA) and differential thermogravimetry (DTG) thermograms of PECONFs. The materials are thermally stable up to a temperature of 400 °C in air. The thermograms demonstrate that mass loss occurs in four steps. The first two steps (mass loss ~20%) below 300 °C are attributed to the desorption of small amounts of water and occluded DMSO (the presence of DMSO was confirmed from the 13 C MAS NMR). Only above 400 °C, continuous mass loss was observed that can be attributed to oxidation and framework decomposition ( Supplementary Fig. S6 ). The mass loss at ~500 °C can be assigned to the oxidation of the organic units. Furthermore, a shoulder was observed at ~700 °C which is due to the decomposition of the P–N units. The TGA thermograms of the samples heated in N 2 environment are shown in Supplementary Figure S7 . All the thermograms show a three-step mass loss with a total mass loss of about 60%. The first two steps were observed below 300 °C and are due to desorption of small amount of water and occluded DMSO. Unlike the sample heated in air, no significant mass loss was observed between 400 to 600 °C. This confirmed that the mass loss at ~500 °C in air is due to the oxidation of the organic units [28] . The materials are thermally stable up to a temperature of 600 °C in N 2 atmosphere. The decomposition of the P-N units did not occur below 800 °C in N 2 . 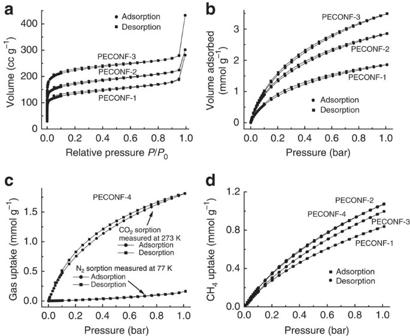Figure 4: Isotherms of PECONF materials. (a) N2and (b) CO2sorption of PECONFs (monolithic form) measured at 77 and 273 K, respectively. N2and CO2uptake increases from PECONF-1 to PECONF-3. (c) N2and CO2sorption isotherms of PECONF-4 monoliths. Due to the absence of macropores, the gas diffusion into the micropores is associated with slow kinetics which leads to a very low N2uptake. (d) Methane sorption isotherms of PECONF-1, PECONF-2, PECONF-3, and PECONF-4 (powder form) measured at 273 K. Isotherms of PECONF-2 and PECONF-4 are very similar and not distinguishable. Gas adsorption To probe for porosity in the PECONFs, we recorded N 2 isotherms of little monolithic pieces (~2–3 mm diameter) at 77 K. Figure 4a shows the N 2 sorption isotherms of PECONF-1, PECONF-2, and PECONF-3. All of these materials show a type-I isotherm, which is typical for microporous materials. The surface area of these samples increases systematically from PECONF-1 to PECONF-3. The Langmuir surface areas were estimated to be 583, 742 and 969 m 2 g −1 for PECONF-1, PECONF-2 and PECONF-3, respectively ( Table 1 ). These values are further comparable with the cumulative surface areas (559, 717, and 939 m 2 g −1 for PECONF-1, PECONF-2 and PECONF-3, respectively) calculated by density functional theory (DFT) & Monte-Carlo analysis ( Table 1 ). The calculated Brunauer–Emmett–Teller surface areas (499, 637, and 851 m 2 g −1 for PECONF-1, PECONF-2 and PECONF-3, respectively) have somewhat lower values compared with the corresponding Langmuir surface areas. The pore volumes estimated at p / p 0 =0.95 are 0.29, 0.35 and 0.43 cm 3 g −1 for PECONF-1, PECONF-2 and PECONF-3, respectively. Details about the physicochemical properties are given in Table 1 . No hysteresis was observed between p / p 0 of 0.40 and 0.85 in these materials confirming the absence of mesopores. The sharp N 2 uptake above p / p 0 =0.95 confirms the macroporosity, which was already seen by TEM and SEM. The isotherms are not completely closed yet at p / p 0 =0.20. A similar non-closed isotherm for a non-crystalline covalent organic framework was recently observed by Hupp et al . [21] Figure 4: Isotherms of PECONF materials. ( a ) N 2 and ( b ) CO 2 sorption of PECONFs (monolithic form) measured at 77 and 273 K, respectively. N 2 and CO 2 uptake increases from PECONF-1 to PECONF-3. ( c ) N 2 and CO 2 sorption isotherms of PECONF-4 monoliths. Due to the absence of macropores, the gas diffusion into the micropores is associated with slow kinetics which leads to a very low N 2 uptake. ( d ) Methane sorption isotherms of PECONF-1, PECONF-2, PECONF-3, and PECONF-4 (powder form) measured at 273 K. Isotherms of PECONF-2 and PECONF-4 are very similar and not distinguishable. Full size image Table 1 Physicochemical properties of PECONF monoliths. Full size table The microporous nature and the high surface area of PENCONF-1, 2, and 3 prompted us to study their CO 2 sorption properties. Figure 4b shows the CO 2 sorption isotherms of PECONF-1, PECONF-2, and PECONF-3 measured at 273 K. For all materials, the CO 2 sorption was completely reversible and no significant hysteresis was observed. The CO 2 uptake of PECONF-1, PECONF-2, and PECONF-3 reaches values of 1.86, 2.85, and 3.49 mmol g −1 , respectively, at 1 atm. The cumulative surface areas calculated from the CO 2 isotherm at 273 K using DFT & Monte-Carlo analysis show values of 438, 670, and 827 m 2 g −1 for PECONF-1, PECONF-2, and PECONF-3, respectively ( Supplementary Table S1 ). These values are somewhat lower compared with the surface areas calculated from the N 2 sorption data of these materials using the Langmuir equation ( Table 1 ). The results indicate that the CO 2 gas uptake scales with the surface area of the material and is inversely proportional to the reactant concentration in the synthesis. PECONF-4 adsorbed only very small amounts of N 2 at 77 K ( Fig. 4c ) and appeared practically non-porous for N 2 . Surprisingly, however, it had a relatively large CO 2 uptake of 1.81 mmol g −1 at 273 K ( Fig. 4c ). The surface area and the pore volume calculated from the CO 2 sorption isotherm of this material using DFT showed values of 433 m 2 g −1 and 0.14 cm 3 g −1 , respectively ( Table 1 ). The CO 2 uptake is remarkable given the small pore volume of only 0.14 mmol g −1 . In fact, PECONF-4 has the highest gas uptake to pore volume ratio of all PECONF materials. The pore size distributions of PECONF-1 to PECONF-4 estimated from the CO 2 sorption using DFT theory are shown in Supplementary Figure S8 . PECONF-1 and PECONF-2 have a narrow monomodal pore size distribution centred on 0.55 nm. PECONF-3 begins to exhibit a bimodal pore-size distribution. PECONF-4 is trimodal with a small additional small maximum is observed at 0.62 nm. The small N 2 uptake in PECONF-4 can be explained by the slow mass transport of N 2 into the strictly microporous PECONF-4 monoliths at 77 K. In contrast, at 273 and 298 K, mass transport is large enough to allow for a significant CO 2 gas uptake in PECONF-4. To confirm that mass transport has an important role in PECONF-4 monoliths, we pulverized PECONF-4 monoliths and remeasured the CO 2 isotherms at 273 and 298 K and the N 2 isotherms at 77 K. As expected, the PECONF-4 material showed at type I N 2 isotherm ( Supplementary Fig. S9 ). The CO 2 capacity increased to a value of 2.95 mmol g −1 ( Supplementary Fig. S10 ). This effect was absent for pulverized forms of PECONF-1, 2, and 3 demonstrating that their hierarchical microporous–macroporous structures provide effective mass transport into the monoliths ( Supplementary Fig. S11 ). We have further studied the methane sorption behaviour of the PECONF materials in powder form. Figure 4d shows the CH 4 sorption isotherms of the PECONF-1 to PECONF-4. All the isotherms are reversible with a high maximum uptake of 1.07 mmol g −1 observed for PECONF-2 and PECONF-4 at 1 bar and 273 K. The PECONF-3 adsorbs a somewhat smaller amount (1.00 mmol g −1 ) of methane. PECONF-1 has the lowest CH 4 gas uptake of 0.83 mmol g −1 . The methane uptake capacities of these samples are still high at 298 K with the maximum uptake of 0.67 mmol g −1 at a pressure of 1 bar observed for PECONF-4. This methane uptake (15 cc g −1 ) is higher compared with the methane sorption (0.8 wt % or 11.1 cc g −1 ) of microporous tris - o -phenylenedioxycyclotriphosphazene van der Waals crystals [34] reported by Sozzani et al . [35] but somewhat smaller than those of covalent organic cages reported by Tozawa et al . [36] However, the latter can only be made by an expensive synthesis procedure. The methane sorption capacities of PECONF-1, PECONF-2, and PECONF-3 are 0.53, 0.63, and 0.58 mmol g −1 , respectively at 298 K ( Supplementary Fig. S12 ). Heats of adsorption To further understand the pore surface characteristics of the materials and the adsorption process, we have calculated the isosteric heats of adsorption ( ΔH ) for CO 2 and CH 4 . ΔH was calculated using the Clausius–Clapeyron equation from the sorption data collected at 273, 298, and 323 K (refs 4 , 37 ). The ΔH value can be obtained from the plot of ln p versus the reciprocal of the temperature. 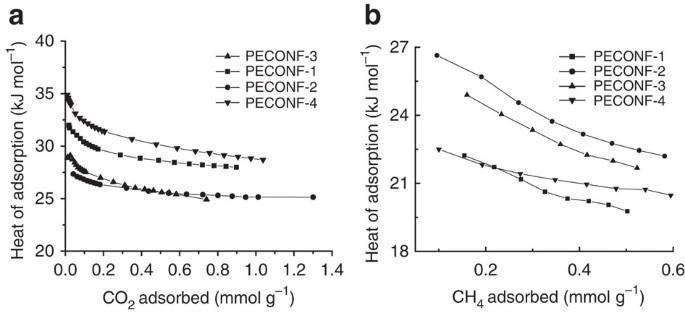Figure 5: Isosteric heat of adsorption of PECONF materials. (a) Isosteric heats of adsorption for CO2(a) and CH4(b) have been calculated from CO2and CH4isotherms collected at 273, 298, and 323 K. Heats of adsorption weakly decrease with increased gas loading. Figure 5a shows ΔH of CO 2 for PECONF-1 to PECONF-4. At the adsorption onset, the ΔH values for PECONF-1, PECONF-2, PECONF-3, and PECONF-4 are 29, 31, 26, and 34 kJ mol −1 , respectively. Remarkably, the isosteric heat of adsorption is nearly independent from the amount of CO 2 adsorbed. The heat of adsorption drops only by 30% (PECONF-2) and 25% (PECONF 3 and 4), respectively. This suggests that if the pore volumes of the materials can be further increased a significantly higher CO 2 gas uptake can probably be achieved even at low CO 2 pressure. Figure 5: Isosteric heat of adsorption of PECONF materials. ( a ) Isosteric heats of adsorption for CO 2 ( a ) and CH 4 ( b ) have been calculated from CO 2 and CH 4 isotherms collected at 273, 298, and 323 K. Heats of adsorption weakly decrease with increased gas loading. Full size image We further calculated the isosteric heat of adsorption of methane for all the samples. Figure 5b shows ΔH of PECONF-1 to PECONF-4. At the adsorption onset, PECONF-1, PECONF-2, PECONF-3, and PECONF-4 show high values of 22, 27, 25, and 22 kJ mol −1 , respectively. The heat of adsorption only weakly decreases with increased methane loading. It is noteworthy, that with the exception of PECONF-4 the methane gas uptake is increasing with increasing heat of adsorption, while the CO 2 gas uptake increases with the surface area. Apparently, in the case of methane adsorption the heat of adsorption is more important than the surface area. The generally high methane uptake for all PECONFs may be explained by H-π interactions. Such interactions have been observed in Van der Waals crystals of tris - o -phenylenedioxycyclotriphosphazene molecules, that are structurally related to the building units of the PECONF materials [35] . Gas selectivity In addition to the high CO 2 uptake and the reversibility, a high selectivity for CO 2 over N 2 is one of the necessary properties for a material to be used as a CO 2 adsorbent. The selectivity for the PECONF monoliths was estimated using the ratios of the Henry law constants [4] . These constants can be calculated from the initial slopes of the isotherms. This method is one of the most common methods to calculate gas selectivities and has been applied extensively to determine gas selectivities of metal–organic frameworks, carbons, and covalent organic frameworks. The calculated CO 2 :N 2 selectivity of PECONF-1 is the highest among the PECONF materials reaching values of 109:1 at 273 K and 51:1 at 298 K ( Supplementary Table S1 ; Supplementary Figs. S13 and S14 ). The value is much higher compared with the next-higher value reported so far (81:1 at 273 K) [4] . Bae et al . [38] reported a CO 2 /N 2 selectivity of 95 at 298 K for a carborane-based metal–organic framework. However, this material appears to be more expensive than our materials. The CO 2 :N 2 selectivities for PECONF-2 ( Supplementary Figs S13 and S15 ) and PECONF-3 ( Supplementary Figs S13 and S16 ) are still high (PECONF-2: 74:1 and 44:1 at 273 and 298 K, PECONF-3: 77:1 and 41:1 at 273 and 298 K). The higher selectivity of PECONF-1 compared with PECONF-2, and 3 can be attributed to its higher heat of adsorption. PECONF-4 has a selectivity of 83:1 and 51:1 at 273 and 298 K, respectively ( Supplementary Figs S13 and S17 ). We further calculated the selectivity of CO 2 :CH 4 and CH 4 :N 2 of these samples at 273 and 298 K ( Supplementary Table S1 ; Supplementary Figs S13-S17 ). PECONF-4 has the highest CO 2 :CH 4 selectivity of 12 at 273 K among all the materials. However, the CH 4 :N 2 selectivity of 16 is maximum for PECONF-1 at 273 K. Sorbents with high selectivity for CH 4 over N 2 are of high practical interest, because methane is often highly diluted by N 2 in natural gas wells. Currently, N 2 /CH 4 separations are still being done cryogenically because of the absence of solid sorbents with high methane sorption capacities and suitable selectivities. To verify the validity of the selectivities estimated from Henry's constant ratios, we have additionally calculated the selectivities by an independent method. We have used ideal adsorbed solution theory (IAST) which allows for the determination of the selectivities as a function of pressure. Because values calculated from Henry constant ratios represent selectivities close to zero pressure, IAST selectivities at zero pressure should match with selectivities calculated from Henry's law constants. Our calculations show that the IAST selectivities are in reasonable agreement with the values obtained from Henry's constant ratios ( Supplementary Figs S18-S23 ). The CO 2 /N 2 selectivity of PECONF-1 at 273 is even somewhat higher (135) compared with the value obtained from Henry's constants (109). It should be noted though that real selectivites can only be determined by measurements that mimic the proposed sorption conditions. For example, in post-combustion CO 2 capture, the contact time with the sorbent would likely to be of the order of seconds; as such, any equilibrium sorption measurements have the potential to be misleading, and in this regard pore size and kinetic mass transport effects are also important. In conclusion, we have synthesized microporous electron-rich covalent organonitridic frameworks in facile condensation reactions from commercially available, relatively inexpensive building blocks. The structures are tunable despite their non-crystallinity and exhibit a remarkable degree of mid-range order. The hierarchical micro-macroporosity is a further advantageous feature of the materials due to the benefits of hierarchical porosity for the mass transport in porous materials. The tunability of the structures translates to their gas sorption properties. The materials adsorb high amounts of CO 2 (up to 3.5 mmol g −1 at 1 atm and 273 K) which is exceeded by only a few other sorbents, namely the amine-functionalized silica MBA-2 (3.8 mmol) [33] , and the amine-functionalized MOFs bio-MOF-11 (6.0 mmol g −1 ), Zn 2 (C 2 O 4 )(C 2 N 4 H 3 ) 2 ·(H 2 O) 0.5 (4.35 mmol g −1 ) [4] , [5] , and Mg/DOBDC (7.2 mmol g −1 ) [39] , [40] . PECONF-1 exhibits one of the highest selectivities (CO 2 over N 2 ) for a sorbent with a reversible CO 2 adsorption–desorption isotherm. The high isosteric heat of adsorption and the high selectivity for CO 2 over N 2 can be explained by Lewis acid–base interactions between the electron-poor CO 2 and the electron-rich sorbent. The heats of adsorption do not decline significantly even at high CO 2 loadings. Similarly, high isosteric heats of adsorption have been observed only for metal-organic frameworks but not for covalent framework materials composed exclusively from non-metals [41] . The strong covalent P–N, N–C, and C–C bonds in the framework provide the materials with high chemical robustness compared with MOFs as seen by the high oxidative stability at temperatures as high as 400 °C. The combination of high thermal and oxidative stability, high gas uptake, low cost, and exceptional selectivity for CO 2 over N 2 make these materials interesting candidates for CO 2 capture applications. Furthermore, the PECONF materials show high sorption capacities and heats of adsorption for methane as well as high selectivities of CH 4 over N 2 which is of high interest for the purification of natural gas that is frequently diluted with N 2 . The mechanically very stable monolithic structure as well as the hierarchical micro-macroporosity suggests further applications, for example in monolithic chromatography. The successful synthesis of the PECONF materials in monolithic shape and the strictly microporous nature of PECONF-4 suggests that this material can also be made as gas-selective membranes. Materials Hexachlorocyclotriphosphazene, Alfa Aesar, 98%. DAB, AK Scientific, 99%. Anhydrous dimethyl sulfoxide (DMSO), Alfa Aesar, 99.8%. Synthesis of PECONFs In a typical synthesis, about 1.5 mmol of DAB and 0.5 mmol of PNC were dissolved in 3, 7.5, 15 and 20 ml of DMSO for the synthesis of PECONF-1, PECONF-2, PECONF-3, and PECONF-4, respectively. The resulting solution was stirred for 30 min at RT. It was then heated at a temperature of 125 °C. Gelation starts as early as 5 min. After 30 min the sample cooled down to room temperature and solid monoliths were collected. All the experiments were carried out in N 2 atmosphere using Schlenk's apparatus. The DMSO from the as-synthesized monoliths was removed by soxhlet extraction using diethyl ether. The obtained solid monoliths were sonicated in 30 ml of water, washed several times with water, and dried in vacuum at 100 °C. The sonicator used in the present research was Cavitator Ultrasonic ME 11 (Mettler Electronics) with a maximum power output of 200 W at 67 kHz. Measurements The microstructures of the specimens were studied by SEM and transmission electron microscopy (TEM). The SEM images of the specimens were taken on a Hitachi S-4300 SEM. The TEM images were taken on a JEOL JEM-2000 electron microscope operated at 200 kV. X-ray diffraction was carried out using a Rigaku Rotaflex diffractometer with a Cu Kα radiation source ( λ =0.15405 nm). The thermogravimetric analysis experiments were carried out both in air and nitrogen using a TA TGA 2950 instrument with a heating rate of 10 °C per minute. 31 P and 13 C CP MAS NMR spectra were obtained at 75.468 MHz on a General Electric NMR Instrument model GN-300 equipped with a Doty Scientific 7 mm MAS probe. 13 C NMR chemical shifts were referenced to the downfield line of adamantine at 38.55 p.p.m., and for 31 P NMR, the chemical shift of 85% H 3 PO 4 was set to zero using external reference standards. The formation of the microporous framework structures were studied by nitrogen and carbon dioxide sorption using an Autosorb-1 instrument (Quantachrome). Before analysis, all the samples were out-gassed overnight at 150 °C in vacuum. The Brunauer–Emmett–Teller surface area analysis was carried out using 5 data points in the pressure range between 0.05 and 0.35 atm. Before IAST calculations, all isotherms were fitted into a Langmuir–Freundlich isotherm. In all cases, a fit >99% was reached. IAST calculations were performed using the software package ChromWorks. How to cite this article: Mohanty, P. et al . Porous covalent electron-rich organonitridic frameworks as highly selective sorbents for methane and carbon dioxide. Nat. Commun. 2:401 doi: 10.1038/ncomms1405 (2011).